Atom-specific spin mapping and buried topological states in a homologous series of topological insulators A topological insulator is a state of quantum matter that, while being an insulator in the bulk, hosts topologically protected electronic states at the surface. These states open the opportunity to realize a number of new applications in spintronics and quantum computing. To take advantage of their peculiar properties, topological insulators should be tuned in such a way that ideal and isolated Dirac cones are located within the topological transport regime without any scattering channels. Here we report ab - initio calculations, spin-resolved photoemission and scanning tunnelling microscopy experiments that demonstrate that the conducting states can effectively tuned within the concept of a homologous series that is formed by the binary chalcogenides (Bi 2 Te 3 , Bi 2 Se 3 and Sb 2 Te 3 ), with the addition of a third element of the group IV. Among the currently known topological insulators (TIs), the layered binary compounds Bi 2 Te 3 , Bi 2 Se 3 and Sb 2 Te 3 have been heavily investigated both experimentally [1] , [2] , [3] , [4] and theoretically [5] , [6] , [7] , [8] , [9] . The realization of many of the predicted topological phenomena requires tuning of the conduction properties of topological insulators, when they are in contact with magnetic semiconductors or superconductors [10] , [11] , [12] , [13] , [14] , [15] , [16] , [17] , [18] , [19] . This tuning or modification of the topological state is usually achieved by doping or intercalation. A promising way to designing new TI materials with tunable surface electronic properties relies on the fact that pseudo-binary systems A IV B VI − m A 2 V B 3 VI (A IV =Ge,Sn,Pb; A V =Bi,Sb; B VI =Te,Se) contain homologous series of ternary compounds. These include a wide variety of mixed-layer materials that have a more complex crystal structure than their parent Bi 2 Te 3 -type compounds. All these systems have tetradymite-like layered structures but with distinct many layered slabs stacked along the c axis of the hexagonal unit cell. The bonding within the slabs is ionic-covalent, whereas the slabs are linked by weak van der Waals forces. 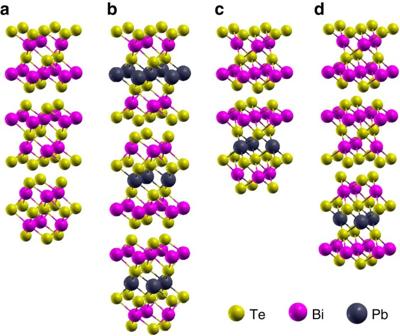Figure 1: Atomic structure of Bi2Te3and Pb-based ternary compoundsnAIVBVImA2VB3VI. (a) Bi2Te3; (b) PbBi2Te4; (c) PbBi4Te7; and (d) PbBi6Te10. The crystal structures of the parent compound and Pb-based systems are shown in Figure 1 . In contrast to Bi 2 Te 3 ( Fig. 1a ), whose structure is formed by quintuple layers (5Ls), the structure of PbBi 2 Te 4 contains septuple layer (7L) slabs ( Fig. 1b ), whereas the rest of compounds in this series are formed by combining 5L and 7L building blocks ( Fig. 1c,d ). Figure 1: Atomic structure of Bi 2 Te 3 and Pb-based ternary compounds n A IV B VI m A 2 V B 3 VI . ( a ) Bi 2 Te 3 ; ( b ) PbBi 2 Te 4 ; ( c ) PbBi 4 Te 7 ; and ( d ) PbBi 6 Te 10 . Full size image In the present paper, we show that most of the A IV B VI − m A 2 V B 3 VI (A IV =Ge,Sn,Pb; A V =Bi,Sb; B VI =Te,Se) compounds are three-dimensional (3D) topological insulators. Peculiarities of bulk spectrum of these materials give rise to more complex surface band structure that depends on surface termination, which can be quintuple- or septuple-layer terminated. We predict the existence of exotic buried topological surface states (SSs) strongly protected against surface perturbations. A layer resolved spin mapping analysis of the topological states indicates layer variations in the spin-helicity and an oscillatory z spin component behaviour in the Dirac cone. We show that the spin localization varies with energy, allowing for control of the spin properties by varying the chemical potential. Parent topological insulators The binary chalcogenides Bi 2 Te 3 , Bi 2 Se 3 , and Sb 2 Te 3 are 3D topological insulators [1] , [2] , [3] , [4] , [5] , [6] , [7] , [8] , [9] with the conducting Dirac SS mostly localized in the outermost 5L block [6] , [9] . 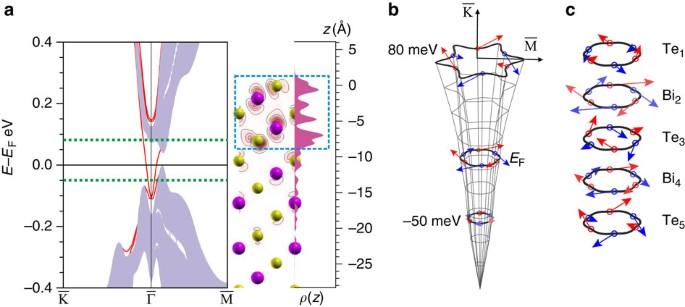Figure 2: Surface electronic and spin structure of the parent Bi2Te3compound. (a) Surface band structure of Bi2Te3and spatial charge density distribution of the Dirac state (blue dashed rectangle marks the outermost 5L block); (b) Dirac cone with iso-energy contours at energies indicated in (a) by green dashed lines and at the Fermi energy; arrows indicate both the total spin magnitude and direction whereas red and blue represent positive and negativeSzcomponent of the spin, respectively; (c) Layer-resolved spin structure of the Dirac state in the topmost 5L of Bi2Te3at the Fermi energy. The surface electronic structure and spatial localization of the Dirac state are shown in Figure 2a for Bi 2 Te 3 as an example. The shapes of the ab-initio iso-energy contours agree very well with those predicted from a model calculation by Fu [20] and are thus expected to show an out-of-plane spin component S z , which increases with increasing warping ( Fig. 2b ). The model predicts a clockwise rotating in-plane spin projection. Our calculations agree with this finding for the subsurface atomic layers of the topmost 5L. However, the rotation direction is reversed at the topmost Te atom Te 1 ( Fig. 2c ). This is similar to the oscillatory layer resolved spin–orbit contributions to the total spin splitting in Pb quantum-well states [21] . Figure 2: Surface electronic and spin structure of the parent Bi 2 Te 3 compound. ( a ) Surface band structure of Bi 2 Te 3 and spatial charge density distribution of the Dirac state (blue dashed rectangle marks the outermost 5L block); ( b ) Dirac cone with iso-energy contours at energies indicated in ( a ) by green dashed lines and at the Fermi energy; arrows indicate both the total spin magnitude and direction whereas red and blue represent positive and negative S z component of the spin, respectively; ( c ) Layer-resolved spin structure of the Dirac state in the topmost 5L of Bi 2 Te 3 at the Fermi energy. Full size image Band structure of the series The Dirac cone in the binary systems originates from the inversion of the bands forming the gap edges: the conventional sequence of the energy levels is inverted by strong spin–orbit coupling (SOC) [22] , [23] . In binary compounds, the bottom of the conduction band in the vicinity of the Γ point is predominantly derived from the states localized at the outermost 5L chalcogen (Te, Se) atoms whereas the top of the valence band is formed by the pnictogen (Bi, Sb) atoms. A similar band inversion is found in PbBi 2 Te 4 , with the only difference that the top of the valence band is occupied by both Bi and Pb ( Fig. 3a ). A more complicated SOC-induced band structure is found in compounds with alternating 5L and 7L slabs, for example PbBi 4 Te 7 ( Fig. 3b ) and PbBi 6 Te 10 ( Fig. 3c ). Here the gap edges can be determined by the states localized on atoms of certain blocks whereas states formed by other blocks lie below or above the gap edges. As will be shown below, this leads to some peculiarities in the formation of the topological state in these compounds. To check the topological character of these materials, we calculated the topological number ν 0 (refs 23 , 24 , 25 ). As all the considered systems have inversion symmetry, we used the method proposed in ref. 23 . Our analysis reveals that most of the considered materials can unambiguously be identified as TIs ( Table 1 ). 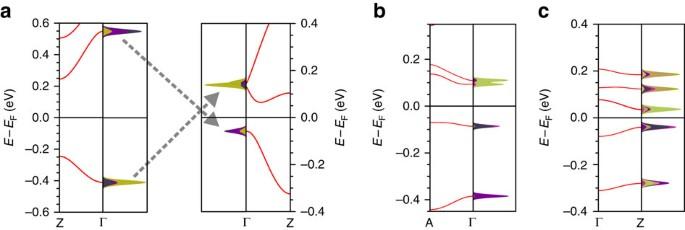Figure 3: Bulk electronic structure of Pb-based ternary compounds in the vicinity of Γ and Z. (a) SOC-induced band inversion scheme in PbBi2Te4. Band structure without SOC-included (left side) and with SOC-included (right side). Black, violet, and green colours in local density of states (LDOS) correspond to Pb, Bi and Te, respectively. Calculated with SOC-included, the orbital composition of nearby gap bands in PbBi4Te7(b) and in PbBi6Te10(c). Black, violet, and pink colours show LDOSs of Pb, and Bi atoms of 5L and 7L blocks, respectively; light green and green correspond to side Te atoms of 5L and 7L blocks in PbBi4Te7, respectively and green, light green, and gold show LDOSs of side Te atoms of 7L block and of 5L block, bordering with other 5L and 7L blocks in PbBi6Te10, respectively. Figure 3: Bulk electronic structure of Pb-based ternary compounds in the vicinity of Γ and Z. ( a ) SOC-induced band inversion scheme in PbBi 2 Te 4 . Band structure without SOC-included (left side) and with SOC-included (right side). Black, violet, and green colours in local density of states (LDOS) correspond to Pb, Bi and Te, respectively. Calculated with SOC-included, the orbital composition of nearby gap bands in PbBi 4 Te 7 ( b ) and in PbBi 6 Te 10 ( c ). Black, violet, and pink colours show LDOSs of Pb, and Bi atoms of 5L and 7L blocks, respectively; light green and green correspond to side Te atoms of 5L and 7L blocks in PbBi 4 Te 7 , respectively and green, light green, and gold show LDOSs of side Te atoms of 7L block and of 5L block, bordering with other 5L and 7L blocks in PbBi 6 Te 10 , respectively. Full size image Table 1 The topological number ν 0 for n A IV B VI · m A 2 V B 3 VI ( n =1; m =1–3) compounds based on Bi 2 Te 3 , Sb 2 Te 3 and Bi 2 Se 3 parent phases. 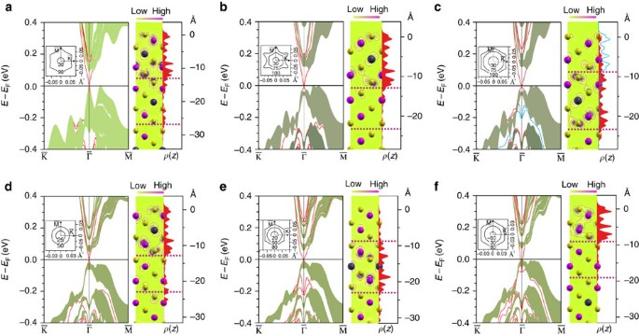Figure 4: Surface electronic structure of Pb-based ternary compounds. Left side of each panel: the calculated surface band structure of Pb-based compounds. The insets show the iso-energy contours of the Dirac cone at various energies. Right side of each panel: spatial distribution of the charge density of the Dirac state at thepoint in theplane and the charge densityρ(z) (red) of this state integrated over the x–y plane;z=0 corresponds to the surface atomic layer. Horizontal dashed lines show boundaries between building blocks. (a) PbBi2Te4; (b) 7L-terminated surface of PbBi4Te7; (c) 5L-terminated surface of PbBi4Te7(the occupied surface state and its in-plane integrated spatial charge density distribution are shown in blue); (d) 7L-terminated surface of PbBi6Te10; (e) 5L-terminated surface of PbBi6Te10; (f) 5–5L-terminated surface of PbBi6Te10. Full size table Surface electronic structure Surface band structures of Pb-Bi-Te and compounds with varying first, second or third elements are given in Figure 4 and Supplementary Figure S1 , respectively. Because the crystal structure of PbBi 4 Te 7 is constituted by alternating 5L and 7L building blocks ( Fig. 1c ), the surfaces formed after cleavage of this crystal have two possible terminations. For the 7L-terminated surface ( Fig. 4b ), the dispersion of the SS is similar to the 5L termination except that the cone is more warped near the conduction band minimum. The spatial distribution of the Dirac state is almost the same as on the PbBi 2 Te 4 surface ( Fig. 4a ); it is localized in the outermost 7L slab. For the 5L-terminated surface ( Fig. 4c ), the situation is more intriguing; the topological SS is also localized in the topmost 7L block, which is now a subsurface block. Thus, in this system, the Dirac state at the point is buried about 10–25 Å under the surface, which makes this state more protected against possible surface modifications. This localization of the Dirac state in the 7L block follows from the aforementioned peculiarity of the bulk band structure of PbBi 4 Te 7 ; as one can see in Figure 3b , the gap edges are formed by spin–orbit inverted states, localized at atoms of the 7L block, which form the Dirac cone on breaking translational symmetry at the surface. Furthermore, at the 5L-terminated surface, the surface states inherent to Bi 2 Te 3 survive, that is, the unoccupied Rashba-type spin-split state and the occupied state at −0.2 eV, which becomes the Dirac state in the parent compound. Accordingly, the dispersion and charge distribution (blue lines in Fig. 4c ) of this state are identical to the Dirac state in Bi 2 Te 3 . Figure 4: Surface electronic structure of Pb-based ternary compounds. Left side of each panel: the calculated surface band structure of Pb-based compounds. The insets show the iso-energy contours of the Dirac cone at various energies. Right side of each panel: spatial distribution of the charge density of the Dirac state at the point in the plane and the charge density ρ ( z ) (red) of this state integrated over the x–y plane; z =0 corresponds to the surface atomic layer. Horizontal dashed lines show boundaries between building blocks. ( a ) PbBi 2 Te 4 ; ( b ) 7L-terminated surface of PbBi 4 Te 7 ; ( c ) 5L-terminated surface of PbBi 4 Te 7 (the occupied surface state and its in-plane integrated spatial charge density distribution are shown in blue); ( d ) 7L-terminated surface of PbBi 6 Te 10 ; ( e ) 5L-terminated surface of PbBi 6 Te 10 ; ( f ) 5–5L-terminated surface of PbBi 6 Te 10 . Full size image This dependence of the electron distribution depth on the surface termination is a general property of such homologous series. For example, the 7L- ( Fig. 4d ) and 5L-terminated ( Fig. 4e ) surfaces of PbBi 6 Te 10 are similar to the corresponding terminations of PbBi 4 Te 7 . Further, the localization of the Dirac state for the two 5L block terminations (5–5L; Fig. 4f ) is similar to that in Bi 2 Te 3 . However, in contrast to the parent system, the SS on this termination forms an exotic cone with a Dirac point in the local gap of the valence bulk band. This unusual behaviour can be understood from the fact that the occupied states localized at the Bi atoms of the 5L block ( Fig. 3c ) are not at the gap edge but below the Bi and Pb states of the 7L block, which for this termination lies deep in the bulk and forms the top of the bulk valence band. 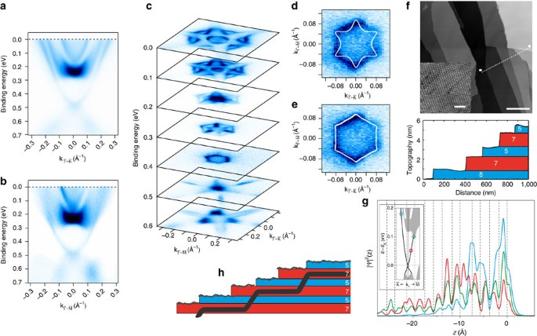Figure 5: ARPES, STM and charge density distribution for PbBi4Te7. Spin-integrated band structure measured along the (a)and (b)directions. Measured iso-energy contours athν=20 eV (c) and comparison between measured and calculated iso-energy contours for the 7-layer (d) and 5-layer (e) surface terminations at 100 meV above the Dirac point. (f) STM topograph showing the mixture of both 5L and 7L steps (bottom) along the dashed line (Vbias= 0.5 V,It=0.25 nA) the white bar is 400 nm. The inset shows an atomic resolution image on a typical 5L layer (Vbias=0.5 V,It=10.5 nA) the white bar is 2 nm. (g) Calculated energy-dependent charge density distribution, the vertical dashed lines indicate the position of the atom cores. (h) Proposed self-protecting behaviour of the topological state. ARPES and STM measurements To study the depth dependence of the SS, we performed high-resolution angle-resolved photoemission spectroscopy (ARPES) and scanning tunnelling microscopy (STM) experiments on PbBi 4 Te 7 single crystals, as shown in Figure 5 . Compared with the ab-initio results from Figure 4b,c , we observe a rigid band shift of about 500 meV, presumably because of bulk and surface defects. Between a binding energy of ~0.3 eV and 0.5 eV, the spectra ( Fig. 5a,b ) and the constant energy contours ( Fig. 5c ) only show the topological surface state. At lower binding energies, one observes both the topological state and the bulk states, which can also be identified by their three-fold intensity symmetry. Along the direction, the bulk bands cross the topological state, whereas along the direction, the topological surface state remains clearly separated from the bulk bands. At binding energies higher than the Dirac point, the topological state and the bulk bands overlap for a small energy range and, for even higher binding energies (from 0.6 eV), one observes only the bulk bands. A detailed analysis of the band dispersion of the Dirac cone, as exemplified by the constant energy contours in Figure 5d,e and the slightly convex energy dispersion, indicates that the photoemission signal primarily originates from a 5L-terminated surface. On the other hand, the STM data in Figure 5f clearly indicate that both surface terminations are present. Images show an alternating step height of 10 Å and 14 Å that corresponds to the predicted height of the 5L and 7L layers of the PbBi 4 Te 7 crystal, respectively. An analysis of surface termination including 18 images with a total area of 212.7 μm 2 reveals a coverage of about 53% for 7L layers and 47% for 5L layers. Atomically resolved images exhibit a clear hexagon lattice. There is no discernible difference between the atomic resolution images of either the 5L or 7L indicating that, in each case, the STM is imaging the tellurium surface sublattice. This apparent contradiction between the ARPES and STM results might be resolved by considering the defect density at the surface and the fact that the topological state lies beneath the surface for energies well below the conduction band ( Fig. 4c ) while on approaching the conduction band it shifts to the outermost 5L block ( Fig. 5g ). The latter fact leads to further increase of the intensity and the linewidth of the Dirac cone at energies at (and above) the conduction band minimum ( Fig. 5a ) with respect to the lower energies due to defect scattering. In the 5L-terminated areas of the surface, the topological state is located for small k || in the 7L subsurface block, protecting this state against scattering at the surface. On the other hand, at the 7L-terminated surface areas defects might push the topological state down to the next subsurface 7L block, as sketched in Figure 5h , where it is no longer accessible by ARPES. This interpretation is corroborated by the absence of the occupied surface state (blue line in Fig. 4c ) in the measurements; the topmost layers can not accommodate a surface state; however, because of its protected nature, the topological state shifts down further into the bulk. This confirms the possibility to grow topological insulators with deep-lying, self-protecting and, thus, technologically relevant surface states. Figure 5: ARPES, STM and charge density distribution for PbBi 4 Te 7 . Spin-integrated band structure measured along the ( a ) and ( b ) directions. Measured iso-energy contours at h ν=20 eV ( c ) and comparison between measured and calculated iso-energy contours for the 7-layer ( d ) and 5-layer ( e ) surface terminations at 100 meV above the Dirac point. ( f ) STM topograph showing the mixture of both 5L and 7L steps (bottom) along the dashed line ( V bias = 0.5 V, I t =0.25 nA) the white bar is 400 nm. The inset shows an atomic resolution image on a typical 5L layer ( V bias =0.5 V, I t =10.5 nA) the white bar is 2 nm. ( g ) Calculated energy-dependent charge density distribution, the vertical dashed lines indicate the position of the atom cores. ( h ) Proposed self-protecting behaviour of the topological state. Full size image Spin-resolved surface band structure After having verified the electronic nature of the topological state, we address its spin structure, which is directly linked to the topological properties. 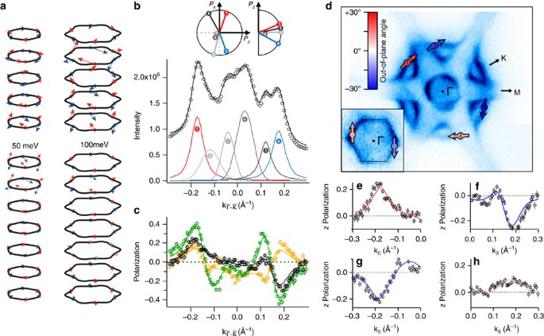Figure 6: Measured and calculated spin texture of PbBi4Te7. (a) Calculated layer-resolved spin structure throughout a complete unit cell at 50 meV and 100 meV above the Dirac point for the 5-layer-terminated surface. (b) Total intensity of a spin-resolved cut 10 meV below the Fermi energy with fitted peaks and the obtained spin polarization vectors where the numbers refer to the fitted peaks. (c) Measured (symbols) and fitted (solid lines) spin polarization along the three spatial directions obtained simultaneously with (b):Pxis orange,Pygreen andPzblack. (d) Summary of the spin texture for two different binding energies (10 meV and 350 meV (inset)), the arrows correspond to the obtained spin polarization vectors where the colour reflects the out-of-plane angle (see colour scale). Out-of-plane polarization spectra and the fits to obtain the polarization vectors corresponding to the numbered crossings in (d), with (e) corresponding to 1, (f) to 2, (g) to 3 and (h) to 4. In Figure 6a , we visualize the calculated layer-resolved spin structure of the Dirac state at 50 and 100 meV above the Dirac point in the two topmost blocks. As one can see, the magnitude of the local spin momentum follows the charge density localization of the state shown in Figure 5g . This behaviour may allow for the possibility to tune the spatial localization of the spin transport channel by shifting the Fermi level. The spin structure of the Dirac state at the 5L-terminated surface of PbBi 4 Te 7 , as well as at the 7L-terminated surface of this compound and at the surfaces of the other Pb-Bi-Te compounds, agrees in all features with that of its parent binary compound. In particular, we find counter-clockwise spin rotation in the topmost Te atom regardless of the surface termination, whereas for all other atomic layers it is clockwise. Figure 6: Measured and calculated spin texture of PbBi 4 Te 7 . ( a ) Calculated layer-resolved spin structure throughout a complete unit cell at 50 meV and 100 meV above the Dirac point for the 5-layer-terminated surface. ( b ) Total intensity of a spin-resolved cut 10 meV below the Fermi energy with fitted peaks and the obtained spin polarization vectors where the numbers refer to the fitted peaks. ( c ) Measured (symbols) and fitted (solid lines) spin polarization along the three spatial directions obtained simultaneously with ( b ): P x is orange, P y green and P z black. ( d ) Summary of the spin texture for two different binding energies (10 meV and 350 meV (inset)), the arrows correspond to the obtained spin polarization vectors where the colour reflects the out-of-plane angle (see colour scale). Out-of-plane polarization spectra and the fits to obtain the polarization vectors corresponding to the numbered crossings in ( d ), with ( e ) corresponding to 1, ( f ) to 2, ( g ) to 3 and ( h ) to 4. Full size image To determine the net helicity for the complete wave function of the Dirac state, we performed spin-resolved ARPES (SARPES) measurements [26] . Figure 6b,c shows a spin-resolved momentum cut along the direction at a binding energy of 10 meV, cutting both through the topological state and the bulk states. By using a vectorial analysis routine [27] , we can assign a three-dimensional spin-polarization vector to each band throughout the constant energy surface, as summarized in Fig. 6d . Even though the exciting photon does not directly couple to the electron spin, the measured polarization does not always directly represent the spin expectation value of the initial state under study due to spin-dependent matrix-element effects. To confirm that the measured spin polarization of the topological surface state is an intrinsic property of the initial state, whereas the polarization of the enclosed bulk bands is induced by the photoemission process, the photon energy dependence of the polarization was studied. Supplementary Figure S3 shows a pair of spin-resolved momentum distribution curve along at the Fermi level measured with 20 eV and 24 eV photon energy. The measured polarization amplitude is strikingly reduced at 24 eV photon energy owing to the larger background as is apparent in the spin-integrated total intensity. Our analysis routine takes the background into account and confirms that neither the direction nor the length of the spin polarization vector of the topological surface state changes significantly on changing the photon energy. On the other hand, the polarization vector of the bulk states is strongly changed as best observed from peaks 2 and 5. The sense of rotation of the topological state is clearly clockwise and the bands are fully polarized, indicating that the spin-eigenstate of PbBi 4 Te 7 corresponds to a positive helicity. The out-of-plane spin polarization shows an even stronger difference in the contributions from each atomic layer, both in direction and magnitude. Unfortunately, SARPES is not suited to link the absolute crystal orientation to the calculations, and it is thus not possible to discriminate which atomic contribution prevails. On the other hand, in the SARPES measurements in Figure 6e–h , the three-fold symmetry of the out-of-plane polarization is reproduced including the smooth changes between . It should be noted that, although the out-of-plane polarization, P z , is related to the warping [28] and disappears when the warping factor goes to zero ( Fig. 2b ), the atomic layer contributions show that warping does not directly determine the direction and magnitude of P z . We have shown that, in the homologous series of ternary compounds based on Bi 2 Te 3 , Bi 2 Se 3 and Sb 2 Te 3 , most of the compounds A IV B VI − m A 2 V B 3 VI (A IV =Ge,Sn,Pb; A V =Bi,Sb; B VI =Te,Se; m =1—3) are 3D topological insulators. Part of these systems ( m =2,3) represent naturally grown superlattices composed of 5L and 7L blocks, which demonstrate much richer physics than the parent TIs. More complex surface electronic and spin structures originate from peculiarities of the bulk spectrum of these materials. Our findings provide a promising pathway to tune both the electronic and spin properties of a topological insulator, by using the ordered ternary compounds on the basis of well-known binary TIs. These compounds exhibit a more complicated surface electronic structure and spin behaviour than their binary parents, which provides an efficient way to manipulate both the spin structure and the spatial localization of the conducting state. This subsequently may allow for a variation of the depth of the spin transport channel below the surface. Our spin-resolved measurements and atomic layer resolved theory provide a new pathway to the aimed design of spin structure properties in topological insulators. Density-functional theory For a complete and reliable description of the electronic structures, we follow a multicode approach, utilizing three different computer codes that are based on density-functional theory. The fundamental quantities are consistently reproduced by all codes. The main part of the electronic structure calculations was performed within the density functional formalism implemented in VASP [29] , [30] . In this plane-wave approach, the interaction between the ion cores and valence electrons was described by the projector augmented-wave method [31] , [32] . To describe the exchange correlation energy, we used the generalized gradient approximation [33] . The Hamiltonian contained scalar-relativistic corrections and the spin–orbit coupling was taken into account by the second variation method [34] . Complementary calculations were performed using the full-potential linearized augmented plane-wave method in thin-film geometry [35] , [36] as implemented in the Fleur-code (URL: http://www.flapw.de ). The atom-resolved spin structures of the topological states were obtained by both VASP and fully relativistic multiple-scattering calculations (layer Korringa–Kohn–Rostoker method) [37] . In the latter case, the Dirac equation is solved from first principles. Experimental lattice parameters were used for calculation of all considered compounds. Crystal growth A single crystalline ingot of PbBi 4 Te 7 was grown from melt by the vertical Bridgman–Stockbarger method. At first, the polycrystalline PbBi 4 Te 7 was synthesized from high-purity (5N) elements in evacuated quartz ampoule at 1,073 K for 8 h mixing incessantly, followed by air cooling. Afterwards, the polycrystalline sample was placed in a conical-bottom quartz ampoule, which was sealed under a vacuum better than 10 −5 Pa. At the beginning of the growing process, the ampoule was held in the hot zone (~955 K) of a specially designed three-zone tube furnace for 24 h for a complete melting of the composition. The charged ampoule moves from the hot zone to the narrow middle zone with the required rate 1.5 mm per hr. The temperature of the middle zone was 855 K corresponding to the crystallization temperature of PbBi 4 Te 7 . Finally, the ampoule entered the third zone of the furnace, where the temperature was 773 K. In this way, layered single crystal with average dimensions of 2 cm in length and 0.7 cm in diameter was obtained. The grown crystal was characterized by X-ray diffraction using a Bruker D8 ADVANCE diffractometer with Cu–K α radiation. The obtained diffractogram confirmed the formation of single-phase PbBi 4 Te 7 crystal that has a hexagonal lattice of the space group P3m1 ( Supplementary Fig. S2 ). By using EVA and TOPAS V3.0 software the unit cell parameters are refined: a =4.418 Å and c =23.948 Å. These parameters are in good agreement with those found in ref. 38 . Scanning tunnelling microscopy Scanning tunnelling microscopy (STM) experiments were performed in an Omicron multichamber UHV-system with a base pressure below 1×10 −10 mbar using a home-built variable temperature scanning tunnelling microscope (VT-STM). Both tungsten-tip and sample were cooled by a Cryovac continuous flow He cryostat to T =30 K. STM topography images were taken in constant current mode at a tunnelling current I t with the bias voltage V bias applied to the sample. Photoemission experiments All photoemission experiments were performed at the Surface and Interface Spectroscopy beamline at the Swiss Light Source at the Paul–Scherrer-Institute using a photon energy of 20 eV. The high-resolution ARPES data was measured at 10 K with a Scienta R4000 hemispherical analyser with a total energy and angular resolution of 12 meV and 0.1 degrees, respectively. The SARPES data was obtained using the COPHEE spectrometer equipped with two orthogonal Mott detectors operated at 40 kV. The spin-resolved data was obtained at 60 K with a total energy and angular resolution of 80 meV and ±0.75 degrees, respectively. How to cite this article: Eremeev, S.V. et al . Atom-specific spin mapping and buried topological states in a homologous series of topological insulators. Nat. Commun. 3:635 doi: 10.1038/ncomms1638 (2012).